Magnetic field-induced dissipation-free state in superconducting nanostructures A superconductor in a magnetic field acquires a finite electrical resistance caused by vortex motion. A quest to immobilize vortices and recover zero resistance at high fields made intense studies of vortex pinning one of the mainstreams of superconducting research. Yet, the decades of efforts resulted in a realization that even promising nanostructures, utilizing vortex matching, cannot withstand high vortex density at large magnetic fields. Here, we report a giant reentrance of vortex pinning induced by increasing magnetic field in a W-based nanowire and a TiN-perforated film densely populated with vortices. We find an extended range of zero resistance with vortex motion arrested by self-induced collective traps. The latter emerge due to order parameter suppression by vortices confined in narrow constrictions by surface superconductivity. Our findings show that geometric restrictions can radically change magnetic properties of superconductors and reverse detrimental effects of magnetic field. In 1936, Schubnikow et al. [1] , [2] broke ground for applications of superconductors. He pointed out the vital distinction between type-I superconductors, in which currents flow only at the surface and superconductivity is destroyed by weak fields and a new type of superconductor, now called a type-II superconductor, capable of carrying bulk supercurrent at relatively high fields. The understanding that the behaviour of type-II superconductors is due to quantized magnetic vortices was achieved by Abrikosov [3] in the 1957. Unluckily, the same vortices that stabilize a superconductor in magnetic fields, compromise its key characteristic, its ability of carrying electrical current with zero resistance. The vortices move in response to an electrical current, dissipating energy and destroying the zero-resistance state [4] . One of the central problems for applications of superconductivity is thus immobilizing vortices to ensure zero electrical power losses. Motivated by this quest, vortex pinning has been over decades the subject of extensive experimental and theoretical studies [5] , [6] , [7] . Generally, the feasibility of superconducting technology is proven. However, it is often desirable to work at temperatures and fields comparable to the critical values where superconductivity is lost. Then, pinning effects are dramatically reduced [7] . Yet there have been alluring communications of an enhancement of superconducting parameters by magnetic field and a negative magnetoresistance in thin superconducting wires [8] , [9] , [10] , [11] . These observations however promising challenged our understanding, as they often referred to the field and temperature range where strong vortex pining were not expected. Here we report a giant reentrance of superconductivity, that is, recovery of the dissipation-free state, by increasing perpendicular magnetic field in a thin wire and thin superconducting film patterned into an array of small holes. We observe suppression of the resistance over at least four orders of magnitude over a wide range of magnetic fields. The experiments are carried out at high magnetic fields and temperatures, where both the wire and the film are densely populated with vortices and where conventional pinning mechanisms are expected to fall ineffective. We demonstrate that this reentrant dissipation-free state forms as a result of constricting vortices into a narrow stripe (in a wire) or small cells (in a film) by surface superconductivity. The densely packed vortices collectively suppress the nearby order parameter thus generating deep potential wells for themselves and self-arresting their own motion. Resistance of wire and perforated film The investigated nanostructures are shown in Fig. 1 . One is a W-based nanowire of the width w =50 nm made through focused-ion-beam-assisted deposition, and the other one is a 5-nm-thin disordered TiN film patterned into an array of holes with a diameter ~120 nm and period a =200 nm. Both systems are extreme type-II superconductors in the dirty limit (ℓ< ξ d (0), with ℓ being the mean free path and ξ d (0) being the superconducting coherence length at zero temperature). In the wire, the superconducting critical temperature is T c =4.3 K and ξ d (0)=6.0 nm. The as-grown continuous film has T c =1.1 K and ξ d (0)=9.3 nm. Shown in Fig. 2a is the magnetic field dependence R ( B ) of the resistance of the W-based nanowire at different temperatures. At T =4 K, R ( B ) dependence is monotonous. At lower temperatures, R ( B ) develops a peculiar N-shape that slightly shifts to higher fields when decreasing temperature. At lowest temperatures, R ( B ) has a maximum and then drops into an extended reentrant zero-resistance region (within the noise level of 100 mΩ, high-field value is of R N =3.56 kΩ). The TiN film data are shown in Fig. 2b . Note that contrasting the wire behaviour, the film remains resistive even at B =0. This occurs because patterning drives the Berezinskii–Kosterlitz–Thouless transition temperature T BKT of the film down to temperatures lower than those of present experiment [12] , and thus unbound vortices and antivortices move freely under the applied current leading to finite resistance. Upon increasing magnetic field, R ( B ) of the film develops a dip around 0.4 T, which again becomes very pronounced at lowest temperatures. At T =0.10 K, the resistance vanishes into the noise over a field range of about 0.7 T (in the interval 0.9/1.35 T and at T =0.1 K, noise level is R =2 mΩ and high-field resistance R ( B =5 T)=200 kΩ, meaning a drop over seven orders of magnitude). The decrease in the resistance is roughly exponential as function of temperature in both systems R exp[ T 0 ( B )/ T ]. The corresponding activation energy T 0 ( B ) is shown in the lower panels of Fig. 2 , and increases by a factor of three with increasing magnetic field. 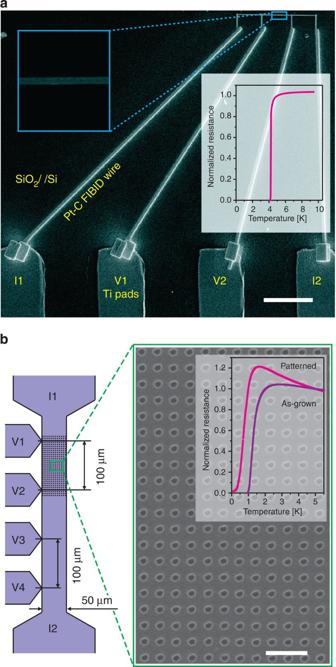Figure 1: Nanopatterned superconducting structures. (a) Scanning electron microscope (SEM) image of a W-based wire grown by FIBID technique on a SiO2/Si substrate. Main panel shows the experimental set-up. The lateral size of the nanowire is 50 nm. Contact pads are made of FIBID Pt-C wires. Scale bar, 5 μm. Left inset displays a zoom of the nanowire and the right inset shows the temperature dependence of the resistance in zero magnetic field normalized to the resistance atT=5 K, which isR=3.56 kΩ. (b) Left: a sketch of the measurement arrangement for the TiN-perforated film. The voltage probesV1–V2 fall within the perforated area, and the probesV3–V4 give a reference from the as-grown continuous film. Right: SEM image of the perforated film, consisting of an array of holes of 120 nm diameter with a period of 200 nm. Scale bar, 500 nm. The inset shows the temperature dependencies of the resistances of the thin film and the perforated film in zero magnetic field normalized to the resistance atT=5 K, which areR=10.87 kΩ for as-grown film, andR=64.93 kΩ for patterned film. Note that, in this case, the resistance does not drop to zero even at the lowest measured temperatures. See Methods for details, andSupplementary Fig. S1for the current dependence, which remains ohmic at low bias. Figure 1: Nanopatterned superconducting structures. ( a ) Scanning electron microscope (SEM) image of a W-based wire grown by FIBID technique on a SiO 2 /Si substrate. Main panel shows the experimental set-up. The lateral size of the nanowire is 50 nm. Contact pads are made of FIBID Pt-C wires. Scale bar, 5 μm. Left inset displays a zoom of the nanowire and the right inset shows the temperature dependence of the resistance in zero magnetic field normalized to the resistance at T =5 K, which is R =3.56 kΩ. ( b ) Left: a sketch of the measurement arrangement for the TiN-perforated film. The voltage probes V 1– V 2 fall within the perforated area, and the probes V 3– V 4 give a reference from the as-grown continuous film. Right: SEM image of the perforated film, consisting of an array of holes of 120 nm diameter with a period of 200 nm. Scale bar, 500 nm. The inset shows the temperature dependencies of the resistances of the thin film and the perforated film in zero magnetic field normalized to the resistance at T =5 K, which are R =10.87 kΩ for as-grown film, and R =64.93 kΩ for patterned film. Note that, in this case, the resistance does not drop to zero even at the lowest measured temperatures. See Methods for details, and Supplementary Fig. S1 for the current dependence, which remains ohmic at low bias. 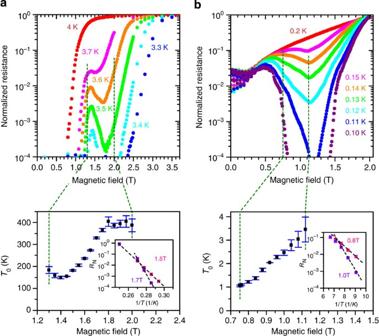Figure 2: Reentrance of the dissipation-free state. (a) The upper panel shows the magnetic field dependences of the resistance of the W-based nanowire taken at different temperatures, the data normalized to high-field values for respective temperatures. Note the large range of fields for reentrant superconductivity. Below 3.5 K, the resistance becomes immeasurably small within nearly half a Tesla. The data atT=3.3 K are normalized to the high-field resistanceRN=3.56 kΩ, the noise level is 100 mΩ, so the overall drop inR(B) in the reentrant region is by the factor 10−4. The lower panel shows the variation of the activation energyT0with the magnetic field in the region of the formation of the reentrant dissipation-free state. Representative Arrhenius plots are given in the inset. (b) The upper panel presents the magnetic field dependences of the resistance of the perforated thin film normalized with respect to the value atB=2 T. AtB<0.5 T, the magnetoresistance shows oscillations with the period ΔB=πħ/(ea2), whereais the pattern unit size. These oscillations are characteristic to weak-link wire networks and are described inSupplementary Fig. S2. At and belowT=0.15 K, the curves develop pronounced V-shape with the position of the minimum almost independent of the temperature. Reentrant superconductivity appears atT=0.11 K, and extends over a field interval of nearly 0.7 T atT=0.1 K. In the region 0.9/1.35 T, the resistance is below the noise level of 2 mΩ. The normalized resistance at 2 T is about 200 kΩ, so that atT=0.1 K, the resistance drops by factor 10−7. We show only four orders of magnitude forR(B) in a logarithmic scale to match the data on a wire. The lower panel shows the growth of the activation energy in the field range corresponding to the ascending branch of the magnetoresistance. The inset demonstrates the representative Arrhenius plots. Error bars in the main bottom panels ofaandbrepresent standard deviations from the linear fit shown in the insets as dashed lines. Full size image Figure 2: Reentrance of the dissipation-free state. ( a ) The upper panel shows the magnetic field dependences of the resistance of the W-based nanowire taken at different temperatures, the data normalized to high-field values for respective temperatures. Note the large range of fields for reentrant superconductivity. Below 3.5 K, the resistance becomes immeasurably small within nearly half a Tesla. The data at T =3.3 K are normalized to the high-field resistance R N =3.56 kΩ, the noise level is 100 mΩ, so the overall drop in R ( B ) in the reentrant region is by the factor 10 −4 . The lower panel shows the variation of the activation energy T 0 with the magnetic field in the region of the formation of the reentrant dissipation-free state. Representative Arrhenius plots are given in the inset. ( b ) The upper panel presents the magnetic field dependences of the resistance of the perforated thin film normalized with respect to the value at B =2 T. At B <0.5 T, the magnetoresistance shows oscillations with the period Δ B = πħ /( ea 2 ), where a is the pattern unit size. These oscillations are characteristic to weak-link wire networks and are described in Supplementary Fig. S2 . At and below T =0.15 K, the curves develop pronounced V-shape with the position of the minimum almost independent of the temperature. Reentrant superconductivity appears at T =0.11 K, and extends over a field interval of nearly 0.7 T at T =0.1 K. In the region 0.9/1.35 T, the resistance is below the noise level of 2 mΩ. The normalized resistance at 2 T is about 200 kΩ, so that at T =0.1 K, the resistance drops by factor 10 −7 . We show only four orders of magnitude for R ( B ) in a logarithmic scale to match the data on a wire. The lower panel shows the growth of the activation energy in the field range corresponding to the ascending branch of the magnetoresistance. The inset demonstrates the representative Arrhenius plots. Error bars in the main bottom panels of a and b represent standard deviations from the linear fit shown in the insets as dashed lines. Full size image Theoretical model: phase diagram To get insight into the mechanism of the observed non-monotonic R ( B ) behaviour and reentrant zero-resistance state, we review the thermodynamics of a superconducting wire (strip) of the width w ξ d . Following the calculations presented in ref. 13 for the slab with the width w ξ d in a parallel field, we deduce the equilibrium phase diagram shown in Fig. 3a . At fields B < B V , the superconducting and normal states are separated by the thermodynamic critical field , with Φ 0 = πħ c / e being the flux quantum [14] . At high fields, B B V , superconductivity vanishes at the upper critical field for surface superconductivity B c3 =1.695 B c2 , where . The field B V divides bulk and surface superconductivity regions: At B < B V =1.61 (Φ 0 / w 2 ), the amplitude of the superconducting order parameter is maximal at the middle line of the wire and is suppressed towards the edges, while at B > B V , the situation is reverse and superconductivity subsists at the surface (edge) sheath [13] , [15] . Equilibrium vortices settle in a strip at B = B V as a one-dimensional vortex row along the median [13] . Within the parameter range of our experiment, the wire accommodates only one vortex row. The point { T V , B V } where B V = B c ( T ) is a tri-critical point. We find in our wire, B V =1.3 T and T V =3.87 K. These values coincide with very good precision with the experimentally found magnetic field of the maximum in R ( T ) ( B max ≈1.4 T) and the experimental temperature above which no maximum is observed (≈3.9 K). Numerical computations of Ginzburg–Landau equations ( Supplementary Discussion and ref. 16 ) illustrate suppression of superconducting order parameter near the middle line and onset of surface-like superconductivity at B > B V ( Fig. 3b ). The temperature above which no vortices appear in the wire (3.8 K) is also in a good agreement with T V , which is also close to temperature defining the condition [17] w >1.85 ξ d ( T ) for vortices to first enter the wire. 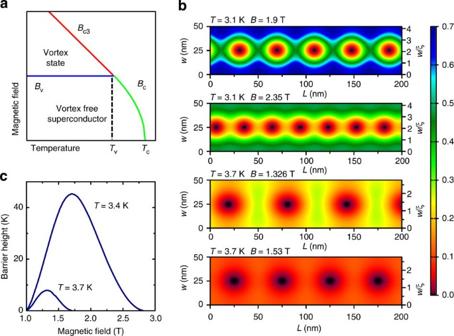Figure 3: Theory for the superconducting wire. (a) Sketch of the phase diagram obtained within the framework of the Ginzburg–Landau description of the superconducting wire withwξ(ref.13). The thermodynamic magnetic fieldBcseparates the vortex-free state from the normal metal atB<BV, atB>BVthe upper-surface critical fieldBc3has this role. WhenBc=BV, we find a tri-critical point in the phase diagram, whose position coincides with the temperatureTVabove which vortices do not enter the wire, because the coherence lengthξdhas grown over the lateral size of the wire. Calculations giveBV=1.4 T andTV=3.9 K for the wire parameters (Fig. 1). (b) Evolution of the order parameter in the superconducting wire with the applied magnetic field. The colour map of the square modulus of the order parameter |Ψ|2for representative temperatures and magnetic fields from numerical solution of the Ginzburg–Landau equations. Colour scale is the same for all four panels. SeeSupplementary Discussionfor details. We use a wire withw=50 nm and material parameters as in the experiment. The upper two panels show the increase in linear vortex density aboveBV. Temperature is too low for vortex motion in the resistance. The two lower panels show, respectively, the order parameter distribution at the magnetic field where barrier height is maximal, that is, close to the minimum of resistance, and close toBc3. (c) The activation barrier for single vortex motion as a function of the magnetic field forT=3.4 and 3.7 K. Non-monotonic behaviour of the barriers reflects the competition between reduced vortex motion, and destruction of superconductivity. The obtained barrier energy is roughly of the same order as the energies discussed inFigs 2and4. Figure 3: Theory for the superconducting wire. ( a ) Sketch of the phase diagram obtained within the framework of the Ginzburg–Landau description of the superconducting wire with w ξ (ref. 13 ). The thermodynamic magnetic field B c separates the vortex-free state from the normal metal at B < B V , at B > B V the upper-surface critical field B c3 has this role. When B c = B V , we find a tri-critical point in the phase diagram, whose position coincides with the temperature T V above which vortices do not enter the wire, because the coherence length ξ d has grown over the lateral size of the wire. Calculations give B V =1.4 T and T V =3.9 K for the wire parameters ( Fig. 1 ). ( b ) Evolution of the order parameter in the superconducting wire with the applied magnetic field. The colour map of the square modulus of the order parameter |Ψ| 2 for representative temperatures and magnetic fields from numerical solution of the Ginzburg–Landau equations. Colour scale is the same for all four panels. See Supplementary Discussion for details. We use a wire with w =50 nm and material parameters as in the experiment. The upper two panels show the increase in linear vortex density above B V . Temperature is too low for vortex motion in the resistance. The two lower panels show, respectively, the order parameter distribution at the magnetic field where barrier height is maximal, that is, close to the minimum of resistance, and close to B c3 . ( c ) The activation barrier for single vortex motion as a function of the magnetic field for T =3.4 and 3.7 K. Non-monotonic behaviour of the barriers reflects the competition between reduced vortex motion, and destruction of superconductivity. The obtained barrier energy is roughly of the same order as the energies discussed in Figs 2 and 4 . Full size image Theoretical model: calculation of the resistance With the phase diagram at hands, we are now equipped to explain the magnetic field dependence of the resistance R ( B ). At B < B V , the dissipation is caused by the ‘external’ vortices crossing the wire. Every vortex sees a dome-like potential barrier with the maximum at the strip median ( Supplementary Discussion and ref. 18 ) and the height linearly decreasing with B . Correspondingly, R exp( B / B *) with B *=0.028 T at T =4 K in a fair agreement with the experimental data. At B = B V , a single row of equilibrium vortices settles in the middle of the wire. Thus, at B > B V the dissipation is governed by the escape of these vortices from the strip across the barriers created by edge superconductivity. At B ≈ B V , the newly established edge barriers are nearly zero. As they also vanish at B = B c3 , where superconductivity is fully suppressed, these barriers must achieve their maximal value at some field between B V and B c3 giving rise to the N-shape of R ( B ) with the maximum at B V . To quantify suppression of R ( B ), we note that as the edge superconducting sheath at B > B V has a width of ~ ξ d , a vortex crossing the edge barrier can be viewed as a phase slip (PS) in the sheath [19] , [20] . To derive the PS activation energy E PS , we employ the concept of the effective resistive medium [21] . There the median band containing vortices can be considered a normal metal with the effective density of normal excitations ν ( B )=( B / B c3 ) ν N , namely the density of excitations within a single core ( ν N ) times the dimensionless linear vortex density ( B / B c3 ). Then the activation energy governing the resistance is the PS nucleation energy, E PS E C ( B ), where is the condensation energy at zero field, Δ is the superconducting gap and is the volume of the PS nucleus ( s =min{ ξ d ( T ), d } and d being the thickness of the sample ( Supplementary Discussion ), and ( B ) is a dimensionless function of the magnetic field such that ( B )~ B / B c3 at B B c3 , and ( B )≈(1− B / B c 3 ) 5/4 at B → B c3 ( Supplementary Discussion and Supplementary Table S1 )). As ( B ) varies from ≈0.15 to 0.4 and E C ( T )≈25 k B T c for the strip, the resistance R ( B ) exp(− E PS / T ) is indeed effectively suppressed over a large field interval between B V and B c3 at T <3.5 K. The remarkable effect of the increase of E PS with the magnetic field reflects the fact that at B B V , the ‘metallicity’ of the resistive central layer of the wire (that is, the effective density of the normal excitations near the median) increases faster than the suppression of surface superconductivity at the edges. The field-induced metallicity means merely an incremental suppression of the order parameter along the median by an increasingly dense vortex chain. Therefore, densely packed vortices dig the more and more deep potential well for themselves with increasing magnetic field and arrest their transverse motion. The current is short circuited by the edge superconducting channels and the wire turns superconducting. Upon further increase of magnetic field, the suppression of edge superconductivity takes over and R ( B ) starts to grow again. That the escape barriers for a vortex chain in the narrow superconducting slab can grow with the magnetic field and lead to enhancement of superconducting parameters was discussed in ref. 22 . Unfortunately, while correctly capturing the trend, the image approach used in ref. 22 did not take into account the collective suppression of the order parameter near the median and thus underestimated the magnitude of the escape barrier. As a result, the effect came out significantly reduced. More precise Ginzburg–Landau simulations accounting for the self-induced suppression of the order parameter along the vortex chain show gigantic increase of the escape barrier with the magnetic field agreeing with the effective medium-based estimates ( Fig. 3b ). Turning to the film, we find the same mechanism of field-promoted metallicity responsible for the reentrant dissipation-free state. As we have already mentioned, the zero-field background resistance results from the free motion of vortices and antivortices, because T BKT (below which they get bound into neutral pairs) is lower than the temperature of our measurements [12] . At B ≲ 0.5 T, the additional vortices induced by the field are trapped in the holes. Accordingly, the order parameter is suppressed around the holes and is maximal within the diamond-like areas between the holes. The perforated film behaves as a weak-link network and the resistance exhibits oscillations on top of the background resistance as a function of the magnetic field [12] ( Supplementary Fig. S1 ), with the period corresponding to integer number of flux quanta per hole. This, so far, is similar to usual ‘vortex-matching effect,’ as seen in the arrays of holes in superconducting films and weak link networks (for example, refs 23 , 24 ). When the amount of vortices in each hole is so large that the currents around holes reach the critical current magnitude, vortices cannot be trapped within holes any more and start to fill the diamond-like areas between them. From this moment, the coherent effects characteristic to weak-link network are suppressed, as evidenced by the disappearance of oscillations in R ( B ). The behaviour of superconductivity surrounding the holes inverts. Vortices piling up in diamond-like cells between the holes suppress the order parameter, which becomes maximal in the rings of width ξ d surrounding the holes. These superconducting rings induce superconductivity in the isthmuses between the holes via the proximity effect and bridge each other to merge into a chain-mail-like network of linked superconducting channels of width ξ d across the film ( Fig. 4 ). The superconducting chain-mail short-circuits the supercurrent across the film similar to edge channels in a wire. The hopping of fluxons between the holes is blocked, as the holes are fully filled up. Vortices clustering in the diamond-like inter-hole cells suppress the nearby order parameter and self arrest themselves. We can understand vortex motion across the superconducting chain mail, which partitions each cell, as phase slips through 1D channels. Each vortex-containing cell can again be described as a resistive effective medium with the effective density of states of normal excitations ν ( B ) ( B / B c3 ) ν N . Note that the diameter of the holes is twelve times ξ d . Thus, as the size of the PS nucleus along the channels is about ξ d , the curvature of chain-mail elements does not change noticeably the PS nucleus energy E PS . One thus expects that the geometric form-factor ( B ), describing the competition between the increasing field-induced metallicity of the resistive parts and the field suppression of surface barriers posed by superconducting channels, is nearly the same for the strip and the film. 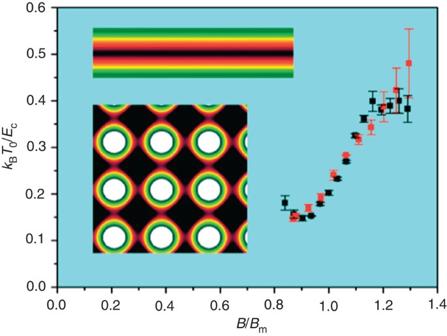Figure 4: Phase slip activation barrier. The experimentally measured activation energy for the descending branch of theR(B) for the superconducting wire (black symbols) and for the perforated thin film (red symbols) in units ofE0(Fig. 2) as a function of the magnetic field normalized to the centre of the magnetic field region where the resistance decreases (between vertical dashed lines inFig. 2). Error bars represent standard deviations from the fit described in the text in relation toFig. 2. The upper panel of the inset shows the nearly tri-layered state leading to recovered superconductivity in a wire. The inner (black) stripe is a nearly metallic state and the green layers show the edge-enhanced superconductivity. The lower inset panel presents corresponding superconducting state in a perforated film. The superconducting annuli surrounding the holes induce superconductivity in the interhole constrictions and results in a chain-mail-like configuration. Figure 4: Phase slip activation barrier. The experimentally measured activation energy for the descending branch of the R ( B ) for the superconducting wire (black symbols) and for the perforated thin film (red symbols) in units of E 0 ( Fig. 2 ) as a function of the magnetic field normalized to the centre of the magnetic field region where the resistance decreases (between vertical dashed lines in Fig. 2 ). Error bars represent standard deviations from the fit described in the text in relation to Fig. 2 . The upper panel of the inset shows the nearly tri-layered state leading to recovered superconductivity in a wire. The inner (black) stripe is a nearly metallic state and the green layers show the edge-enhanced superconductivity. The lower inset panel presents corresponding superconducting state in a perforated film. The superconducting annuli surrounding the holes induce superconductivity in the interhole constrictions and results in a chain-mail-like configuration. Full size image To establish that the mechanism of reentrant superconductivity is unique, we plot in Fig. 4 the measured activation barriers at the descending branches of R ( B ) for both the nanowire and the film, normalized to their respective nucleus energies E C (reflecting specific properties of each material), as a function of the normalized magnetic field B / B min . For the nanowire E C / k B =101.3 K at T =3.2 K, and E C / k B =7.18 K for the film at T =0.12 K. Both curves collapse on top of each other evidencing the universal character of the F ( B ) function and thus, the common mechanism for the reentrance of the dissipation-free state in a strip and a patterned film. We have demonstrated giant magnetic field-induced reentrant superconductivity in two seemingly disparate systems, a thin W-based wire and thin TiN film patterned into an array of holes. By juxtaposing their respective R ( B ) behaviours and system parameters, we have revealed the underlying mechanism of the effect. The giant reentrance rests on two components. The first is that surface (edge) superconductivity arrests vortex motion by constricting them into immobile aggregates: the denser the vortex cluster, the better the superconducting order parameter around this cluster is suppressed and the deeper the self-generated potential well confining vortices. The effective resistive medium grows more metallic with field. The density of normal excitation states is proportional to B , and so does the energy of the PS nucleus. Thus, increasing magnetic field suppresses the phase slips across the edge superconducting channels until the suppression of surface superconductivity itself prevails. The second component is the specific geometry ensuring that the volume occupied by edge superconducting channels is comparable to that of the vortex-carrying resistive medium. In that case, collective depinning effects do not develop, implying that the surface barrier for vortex escape can stand applied currents comparable to the pair-breaking current. Our findings open new routes to design superconducting devices working at high magnetic fields and temperatures, and mark an important step towards resolving the long-standing problem of extending the coherent dissipation-free superconducting state to high field and temperature range. Fabrication and characterization of the wire Amorphous W-based superconducting nanowires were grown by the focused ion beam-induced deposition (FIBID) technique in a dual beam, Nova 200 Nanolab (FEI Company) equipment. FIBID consists in the local growth of nanostructures on a substrate where the suitable precursor gas molecules are adsorbed and dissociated by the focused ion beam (FIB) [25] . The technique can be viewed as a local chemical vapour deposition method induced by the FIB. The typical lateral size and the thickness obtained using the FIBID range from few nanometres to several micrometres, and, under appropriate conditions described below, the superconducting nanostructures can be obtained. As FIBID is a direct-write technique, it does not involve the succession of complex procedures needed to make other superconducting nanostructures, such as electrochemical deposition or carbon nanotube templates, which have been used in the past to create small superconducting wires [26] . We were using the Ga-based FIB in combination with the precursor gas W(CO) 6 . It has been shown that the resulting deposit is superconducting with T c around 5 K (ref. 27 ). The precursor gas was injected into the process chamber by means of a needle inserted in the vicinity of the specimen, around 50 μm away in x – y direction and around 150 μm away in the z direction of the substrate surface. This allows for an efficient FIBID process. A silicon wafer with the 250-nm thermally grown oxide layer was used as a substrate. The nanowire was grown in the geometry shown in Fig. 1 , having four pads made of the same material as the nanowire itself. At the first stage, a horizontal nanowire of the 8-μm length and four perpendicular equidistant nanowires of the 2-μm length, used for the I1, V1, V2 and I2 connexions, were deposited. The used FIBID parameters were as follows: the ion beam acceleration voltage was 30 kV; the ion beam current was 1 pA; the dwell time was 200 ns; the scanning pitch was 10.5 nm; the chamber base pressure was 1 × 10 −6 mbar; the chamber pressure during FIBID was 6 × 10 −6 mbar; and the precursor temperature was 55 °C. The in situ scanning electron microscope images shown in Fig. 1 were performed by the same equipment using a field-emission electron gun, thus providing high-resolution images of the nanowires and giving a good determination of the lateral size (50 nm). Additionally, we made atomic force microscopy measurements, giving a good thickness uniformity (30 nm with a maximum variation of ±5 nm) along the length of nanowires [28] . The set-up for performing measurements on the nanowire is shown in Fig. 1 . The Pt-C wire was grown by FIBID on the top of the four small paths of the nanowire (using (CH 3 ) 3 Pt(CpCH 3 ) as the precursor gas), connecting the nanowire to Ti pads where aluminium wires could be bonded. The Ti pads were made using the optical lithography lift-off method and e-beam evaporation with a thickness of 150 nm. More details of the contacting method are given in refs 28 , 29 . Magnetotransport measurements were performed using a commercial Physical Properties Measurements System (PPMS from Quantum Design) in the temperature range from 300 K down to 2 K. The magnetic field was applied perpendicular to the substrate and the ac measurement mode was used. The composition of the W-based FIBID nanostructures in atomic percentages are as follows. The W percentage: 40±7%; C percentage: 43±4%, Ga percentage: 10±3%, O percentage: 7±2%. The composition remains the same through the full thickness [30] . Superconducting properties of the W-based FIBID thin films of equal composition and the same growth methods have been previously studied in refs 30 , 31 . The classical vortex lattice behaviour was found, with B c2 ( T ) following a clear mean field behaviour [30] . The Ginzburg–Landau parameters were calculated from the normal resistance of 2.75 μΩm and the derivative of upper critical field at T c , namely (d B c2 /d T )( T = T c )=2 T K −1 , resulting in ξ (0)=6 nm, λ (0)=640 nm, and the GL parameter κ = λ (0)/1.63 ξ (0)=65. The thermodynamic critical field is B c =40 mT, the upper critical magnetic field B c2 =6.5 T and the superconducting gap is Δ 0 =0.66 meV. A neat Abrikosov hexagonal vortex lattice was observed in the films through scanning tunneling microscopy and spectroscopy (STM/S) [30] , [31] . The material parameters inferred from the data are as follows: the diffusion coefficient D =0.51 cm s −1 , R □ =59.3 Ω, and the density of normal excitation states ν = σ /( e 2 D )≡1/( e 2 DR □ d )=4.3 × 10 47 J −1 m −3 . Fabrication and characterization of the perforated film. A smooth, continuous and uniform TiN film with the thickness of 5 nm was synthesized by atomic layer deposition on a SiO 2 /Si substrate at the deposition temperature T d =350 °C. High-resolution transmission electron microscopy was performed using a JEOL-4000EX (Japan) microscope operated at 400 keV. Electron transmission micrographs and diffraction patterns revealed the polycrystalline structure with the densely packed crystallites ( Supplementary Fig. S2 ) (the average grain size is about 5 nm). The cross-section micrograph of the film ( Supplementary Fig. S2c ) shows the atomically smooth interface between the SiO 2 substrate and the TiN film and the atomically smooth surface of the TiN film. To carry out the transport measurements the film was first patterned by means of the conventional UV lithography and plasma etching into the bridges 50 μm wide and with the 100 μm distance between the voltage probes ( Fig. 1b ). Then, making use of the electron lithography and the subsequent plasma etching, a square lattice of holes with the diameter ~120 nm and the period a =200 nm covering the 50 × 120 μm 2 area, was created ( Fig. 1b ). The voltage probes V1–V2 were designed to fall within the nanopatterned domain of the film, while the probes V3–V4 were placed within its continuous (non-patterned) section to measure thus the resistance of the original continuous film. The nanopatterned section of the film confined between the probes V1–V2 contained 50 μm × 100 μm/(200 nm) 2 =125,000 elemental units. As a first step of the electron lithography process, the films were spin-coated with the poly(methyl methacrylate) (PMMA) electron-beam resist with the molecular weight 950.000 diluted with anisole, providing the thickness of 180 nm after 30 s spinning at 3,000 rpm. The samples coated with PMMA were subsequently baked over 30 min in convection oven at the temperature 170 °C. The desired network pattern was created by the exposure of the PMMA layer to the electron beam using Raith 150 high-resolution electron-beam lithography system (the diameter of the beam is of about 2.4 nm at 20 kV). The PMMA was used as a positive electron-beam resist, as it provides high contrast with respect to further developing. Upon removing of the exposed parts of the PMMA by the standard methyl-isobutyl-ketone (MIBK)–isopropyl 1:3 solution, the pattern mask have got formed. Usually in the electron-beam lithography systems the dots are designed as an array of single elements with the quantity equal to the quantity of dots. Then the time necessary for settling the unique element gets critical for the overall time of the structure exposure. To design our TiN-nanopatterned samples, we have developed a method, which allows the exposure of the array of 10 9 dots over the time as short as a few tenths of minutes. The strategy of method was to write a large rectangle, using a step equal to the array step. The size of dots depended on the area dose and could be varied from 20 nm up to 120 nm as a result of the Gaussian shape of electron beam and of the proximity effect. We have determined that the best patterning results are achieved if the energies of the electrons in the beam exceed or are equal to 20 kV, and the apertures size are small enough, about 7.5 μm, to ensure the round shape of dots. The chosen design (pairs of V1–V2 and V3–V4 probes) allows comparing the physical properties of the patterned sections, the non-patterned sections of the film that were subject to whole procedure except for being exposed to electron beam and the films that were not subject to the electron-beam lithography process at all. The superconducting and transport properties of the second and the latter appeared the same, proving thus that the electron-beam lithography treatment did not damage the TiN films and remained identical to the films that were fully characterized by the infrared [32] , sample D15 and low-temperature scanning tunnelling spectroscopy [33] , [34] , sample TiN2. The temperature T and the magnetic field B dependences of the resistance were measured using the standard four-probe low-frequency ac techniques at the frequency 1 Hz with an ac current 0.3 nA. So the current was sufficiently small to ensure the linear response regime as was verified by direct measurements of the current–voltage ( I – V ) characteristics ( Supplementay Fig. S1b ). The magnetic field was applied perpendicular to the film surface. Transport and superconducting properties of our sample are close to those used in earlier studies [12] , [35] . The sample parameters are as follows: the diffusion constant D =0.32 cm 2 s −1 , the superconducting coherence length ξ (0)=9.3 nm, the transition temperature, T c =1.115 K, λ (0)=2.4 μm, κ =158 and the superconducting gap Δ=0.22 meV. Further, using the TiN film room temperature resistance per square R □ =( e 2 Dνd ) −1 =2.94 kΩ, we estimate the density of states as ν =8.3 × 10 46 J −1 m −3 . Shown in the Supplementary Fig. S1 are the data on the transport measurements of the TiN-based perforated film. Supplementary Figure S1a displays oscillations of the magnetoresistance observed in the range B <0.5 T up to temperatures 0.7 K evidencing the existence of the superconducting order parameter in the temperature range in question. These oscillations are characteristic to 2D Josephson junction arrays, proximity-effect junction arrays and superconducting wire networks, and reflect the collective behaviour and effect of synchronization of the Josephson phases in 2D multiconnected superconducting systems, for detailed discussion see ref. 35 . Supplementary Figure S1b shows the I – V characteristic in a log–log scale and the inset presents the same data as the differential resistance d V /d I versus I plot at zero magnetic field and T =0.1 K. Using the magnitude of the critical current evaluated from the position of the maximum of the d V /d I versus I curve [35] , we have determined the critical current through the whole network I c =0.17 μA, yielding the critical current i c =0.68 nA per one constriction. Having determined the critical current, one estimates the Pearl penetration depth λ ⊥ = ħ /(2 eμ 0 i c )=38 cm, and the Josephson coupling E j =( ħ i c /2 e ). It yields E j / k B 0.016 K, and, accordingly, T BKT = πE J /(2 k B ) 0.025 K. How to cite this article: Córdoba, R. et al. Magnetic field-induced dissipation-free state in superconducting nanostructures. Nat. Commun. 4:1437 doi: 10.1038/ncomms2437 (2013).